Regulation ofArabidopsisphotoreceptor CRY2 by two distinct E3 ubiquitin ligases Cryptochromes (CRYs) are photoreceptors or components of the molecular clock in various evolutionary lineages, and they are commonly regulated by polyubiquitination and proteolysis. Multiple E3 ubiquitin ligases regulate CRYs in animal models, and previous genetics study also suggest existence of multiple E3 ubiquitin ligases for plant CRYs. However, only one E3 ligase, Cul4 COP1/SPAs , has been reported for plant CRYs so far. Here we show that Cul3 LRBs is the second E3 ligase of CRY2 in Arabidopsis . We demonstrate the blue light-specific and CRY-dependent activity of LRBs (Light-Response Bric-a-Brack/Tramtrack/Broad 1, 2 & 3) in blue-light regulation of hypocotyl elongation. LRBs physically interact with photoexcited and phosphorylated CRY2, at the CCE domain of CRY2, to facilitate polyubiquitination and degradation of CRY2 in response to blue light. We propose that Cul4 COP1/SPAs and Cul3 LRBs E3 ligases interact with CRY2 via different structure elements to regulate the abundance of CRY2 photoreceptor under different light conditions, facilitating optimal photoresponses of plants grown in nature. CRYs are photolyase-like flavoproteins that act as photoreceptors in plants or core components of the molecular clock in mammals [1] , [2] , [3] . Regulation of CRY abundance is an important mechanism to control cellular photo-responses and chrono-responses. For example, two cullin 1 family E3 ubiquitin ligases, SCF FBXL3 and SCF FBXL21 , regulate ubiquitination and degradation of mCRYs to govern the circadian clock in mammals [4] , [5] , [6] , [7] , [8] . Similarly, a cullin 1-based E3 ubiquitin ligase receptor, Jetlag, and a cullin 4-based E3 ubiquitin ligase receptor, Brwd3, bind to dCRY to regulate ubiquitination of Tim (Timeless) and dCRY in Drosophila [9] , [10] . Arabidopsis cryptochrome 2 (CRY2) is one of the best studied plant CRYs that mediate blue light inhibition of cell elongation and photoperiodic promotion of floral initiation [11] , [12] . These physiological activities of CRY2 are regulated by at least three blue light-dependent mechanisms. First, CRY2 undergoes blue light-dependent oligomerization to become active tetramers [13] , [14] , [15] , [16] , [17] . The BIC1 and BIC2 (Blue-light Inhibitors of Cryptochromes 1 and 2) proteins interact with photoexcited CRY2 to negatively regulate CRY2 photooligomerization in light, whereas the active CRY2 homooligomers may also undergo thermal relaxation to become inactive monomers in the absence of light [14] , [15] , [16] , [17] . Second, the activity of CRY2 homooligomers are positively regulated by protein phosphorylation reactions catalyzed by four related protein kinases PPKs (Photoregulatory Protein Kinases 1–4) [18] , [19] , [20] . Third, the photoexcited and phosphorylated CRY2 proteins undergo polyubiquitination catalyzed by the E3 ubiquitin ligase Cul4 COP1/SPAs and subsequently degraded by the 26S proteasome [11] , [21] , [22] . Like animal CRYs, the abundance and overall cellular activity of plant CRYs are regulated by phosphorylation, ubiquitination, and proteolysis [3] . However, only a cullin 4 family E3 ubiquitin ligase, Cul4 COP1/SPAs , is presently known to regulate ubiquitination and degradation of plant CRYs [3] , raising the question how the highly conserved CRYs are differentially regulated in different evolutionary lineages. Under natural light conditions, plants rely on the coaction of blue light receptors CRYs and the red/far-red light receptors phytochromes phys [23] , [24] to achieve the optimal photoresponses [25] . Mechanistically, the CRY-phy coaction could be achieved by different photoreceptors physically complexing with the same signaling proteins, such as bHLH transcription factors, Phytochrome Interacting Factors (PIF1-8) [26] , Photoregulatory Protein Kinases (PPK1-4) [20] , [27] , the substrate receptors and co-receptors of the Cul4 COP1/SPAs E3 ligases, COP1 [28] and SPAs [29] . For example, CRY2 interacts with PPKs, which catalyze blue light-dependent phosphorylation of CRY2 to positively regulate the functions, polyubiquitination, and degradation of CRY2 [20] . On the other hand, PPKs interact with the phyB-PIF3 complex to negatively regulate the function of phyB by the so-called “mutually assured destruction” mechanism [27] , [30] . According to this hypothesis, the photoexcited phyB interacts with PIF3, recruiting PPKs to phosphorylate PIF3; phosphorylated PIF3 interacts with the substrate receptors of the Cul3 LRBs , Light-Response Bric-a-Brack/Tramtrack/Broad (LRB 1-3), which are the substrate receptors of the Cul3 LRBs E3 ligases that catalyze polyubiquitination and degradation of PIF3 that also leads to phyB degradation [27] . Arabidopsis genome encodes three LRBs, LRB1, LRB2, and LRB3 [30] , [31] . LRB1 and LRB2 share higher homology and higher levels of mRNA expression than LRB3, and they act redundantly to suppress phyB-dependent photoresponses [31] . It remains unclear whether Cul3 LRBs play roles in the CRY-dependent signaling process in addition to its important function regulating PIF3 ubiquitination and phyB-dependent red-light responses. LRBs are required for the CRY-dependent blue light responses We have previously shown that the blue light-dependent ubiquitination and proteolysis of CRY2 is diminished but not completely abolished in the cop1 null mutant [22] , suggesting the existence of another E3 ubiquitin ligase in addition to Cul4 COP1/SPAs . 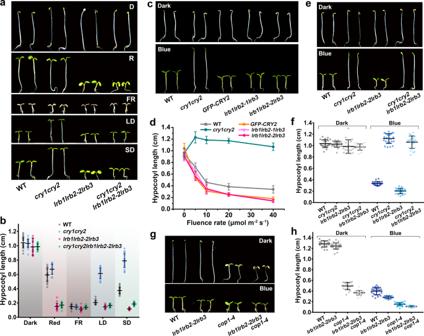Fig. 1: LRBs are required for blue light responses. a6-day-old seedlings grown in darkness (D), red light (R, 20 μmol m−2s−1), far-red light (FR, 6 μmol m−2s−1), long days (LD, 16 h light / 8 h dark), or short days (SD, 8 h light / 16 h dark).bMeasurements of hypocotyl length of seedlings shown in (a), (mean ± SD).c6-day-old seedlings grown in darkness or blue light (10 μmol m−2s−1).dMeasurements of hypocotyl length of indicated genotypes grown under blue light of different intensities (0, 5, 10, 20, and 40 μmol m−2s−1) for 6 days, (mean ± SD,n= 25).e,g6-day old seedlings grown in darkness or blue light (20 μmol m−2s−1).f,hMeasurements of hypocotyl length of seedlings shown in (e) and (g), (mean ± SD). The above experiments were repeated at least three times with similar results. We analyzed CRY2 complexomes isolated from transgenic Arabidopsis plants overexpressing GFP-CRY2, using the immunoprecipitation-mass spectrometry (IP-MS) [20] , and identified LRB1 and LRB2 as CRY2-associated proteins in a blue light-dependent manner (Supplementary Table 1 ). We analyzed flowering time of the lrb1lrb2-2lrb3 triple mutant. The lrb123 triple mutant showed slightly delayed flowering in long day, and it appears somewhat additive to the delay-flowering of the cry1cry2 mutant (Supplementary Fig. 1 ). However, given the known role of LRBs as regulators of phytochrome abundance and functions [30] , [31] , and the antagonistic as well as redundant functions of phytochromes and cryptochromes in the control of flowering time [3] , it is technically difficult to clarify the exact roles of LRBs in the CRY-dependent control of flowering-time by only the genetic analyses. We then examined whether LRBs play a role in blue light-dependent regulation of seedling development. As reported previously [30] , the lrb123 triple mutant showed no apparent abnormality when grown in darkness or far-red light, but it exhibited a dramatic short-hypocotyl phenotype when grown in continuous red light (Fig. 1a, b ). The lrb123 triple mutant also showed short-hypocotyl phenotype when grown in either long-day or short-day photoperiods illuminated with white light (Fig. 1a, b ). These results are consistent with the established function of LRBs regulating red light-dependent activities of phyB [30] , [31] . When grown in continuous blue light, the cry1cry2 mutant developed long hypocotyl phenotype as previously reported [32] , whereas the lrb123 showed hypocotyls modestly shorter than that of the wild-type seedings (Fig. 1c, d ). The short hypocotyl phenotype of lrb123 mutant in blue light can be rescued by constitutively overexpressing the LRB2 protein in the lrb123 mutant (Supplementary Fig. 2 ). This defective phenotype of the lrb123 mutant seedlings (6-day-old) is more apparent in seedlings grown in blue light of the light intensities higher than 10 μmol m −2 s −1 (Fig. 1d ), which is consistent with the previous report that showed hardly distinguished phenotype of the wild-type and the lrb12 double mutant (4-day-old) grown in continuous blue light with the light intensities of 10 μmol m −2 s −1 or lower [31] . These results argue for a light intensity-dependent function of LRBs in blue light. To examine the functional relationship between CRYs and LRBs, we prepared the cry1cry2lrb123 quintuple mutant and compared the hypocotyl phenotype of the quintuple mutant with its parents (Fig. 1e, f ). When grown under continuous blue light, the cry1cry2 mutant and the lrb123 mutant exhibit long or short hypocotyl phenotype, respectively. However, the cry1cry2lrb123 quintuple mutant shows the long hypocotyl phenotype indistinguishable from that of the cry1cry2 mutant parent in blue light (Fig. 1e, f ), but not in other light conditions (Fig. 1a, b ). This result demonstrates that the function of LRBs in blue light is dependent on the activity of the blue-light receptor CRYs. Comparing with the lrb123 parent, the lrb123cop1 quadruple mutant shows de-etiolated phenotype of the cop1 parent in darkness but a slight additive effect of the lrb123 and cop1 mutants in blue light (Fig. 1g, h ). Taken together, these results argue that LRBs regulate plant development by controlling not only the red light-dependent activity of phytochromes but also the blue light-dependent activity of cryptochromes. Fig. 1: LRBs are required for blue light responses. a 6-day-old seedlings grown in darkness (D), red light (R, 20 μmol m − 2 s −1 ), far-red light (FR, 6 μmol m −2 s −1 ), long days (LD, 16 h light / 8 h dark), or short days (SD, 8 h light / 16 h dark). b Measurements of hypocotyl length of seedlings shown in ( a ), (mean ± SD). c 6-day-old seedlings grown in darkness or blue light (10 μmol m −2 s −1 ). d Measurements of hypocotyl length of indicated genotypes grown under blue light of different intensities (0, 5, 10, 20, and 40 μmol m −2 s −1 ) for 6 days, (mean ± SD, n = 25). e , g 6-day old seedlings grown in darkness or blue light (20 μmol m −2 s −1 ). f , h Measurements of hypocotyl length of seedlings shown in ( e ) and ( g ), (mean ± SD). The above experiments were repeated at least three times with similar results. Full size image LRBs are required for the blue light-dependent CRY2 degradation We next tested how LRBs regulate cryptochrome activity by examining the blue light-dependent degradation of CRY2 in the lrb123 mutants. Results shown in Fig. 2 demonstrate that LRBs are required for the blue light-induced degradation of CRY2. The CRY2 protein level decreased by at least 70% (in 30 min) to 85% (in 60 min) in etiolated wild-type seedlings transferred to blue light (30 μmol m −2 s −1 ) (Fig. 2a, b ). In contrast, levels of the CRY2 protein exhibited little change in one lrb123 triple mutant allele ( lrb1lrb2-1lrb3 ) or <50% decrease in the second lrb123 triple mutant allele ( lrb1lrb2-2lrb3 ) under the same condition (Fig. 2a, b ). This result indicates that lrb1lrb2-1lrb3 is a slightly stronger allele in comparison to lrb1lrb2-2lrb3 . We next compared the blue light-induced CRY2 degradation in lrb123 , cop1 , and lrb123cop1 quadruple mutant in seedlings grown in continuous dark or blue light. CRY2 shows similar abundance in the wild-type and both lrb123 triple mutant alleles grown in continuous blue light, whereas the level of CRY2 is higher than that of the wild-type in the cop1 mutant grown in continuous blue light (Fig. 2c, d ). Results of this experiment indicate that COP1, but not LRBs, determines abundance of the CRY2 protein in seedlings exposed to prolonged blue light. We hypothesize that LRBs are responsible for the rapid blue light response of CRY2 proteolysis but not the prolonged photoresponse of CRY2 proteolysis, whereas COP1 is required for the prolonged photoresponse of CRY2 proteolysis. This difference may be explained, at least partially, by the respective roles of Cul3 LRBs and Cul4 COP1/SPAs ligases in CRY2 signal transduction. COP1 is a major signaling molecule of CRY2 [33] , [34] , [35] , in addition to its role as a E3 ligase of CRY2 [18] , but LRBs are not known to play a direct role in the CRY2 signaling transduction. It is conceivable that the CRY2 suppression of COP1 activity in the early stage of light exposure, including COP1-dependent CRY2 ubiquitination, may be partially overcome by some feedback regulations during prolonged light exposure. We further tested the hypothesis that LRBs and COP1 may regulate CRY2 degradation under different light conditions, by comparing the photoresponsive CRY2 proteolysis in etiolated seedlings transferred to blue light from 30 min to 14 h (Fig. 2e, f ). In etiolated seedlings exposed to blue light, CRY2 degradation shows clear defect in the lrb123 triple mutants within 2 h of light exposure, but the cop1 mutant exhibits more pronounced defect in CRY2 degradation during prolonged light exposure. These results are consistent with the observations that more CRY2 accumulated in the cop1 mutant in continuous blue light, but not in the lrb123 mutant alleles (Fig. 2c, d ). Importantly, little CRY2 degradation was detected in the lrb123cop1 quadruple mutant for both short or long exposure of blue light (Fig. 2c–f ). We concluded that LRBs and COP1 are both required for the blue light-induced CRY2 degradation. Fig. 2: LRBs and COP1 regulate the rapid or prolonged proteolysis of CRY2, respectively. a Representative immunoblots showing the abundance of endogenous CRY2 in the 7-day-old etiolated wild type (WT) and lrb123 mutants irradiated with 30 μmol m −2 s −1 of blue light for the indicated time. b Quantitative analysis of CRY2 abundance from immunoblots shown in ( a ). Data are presented as mean ± SD ( n = 3 individual immunoblots). c Representative immunoblots showing the abundance of endogenous CRY2 in seedlings of indicated genotypes grown in darkness (D) or continuous blue light (cB, 30 μmol m −2 s −1 ). d Quantitative analysis of CRY2 abundance from immunoblots shown in ( c ). Data are presented as mean ± SD ( n = 3 individual immunoblots). e Representative immunoblots showing degradation of the endogenous CRY2 in 7-day-old etiolated seedlings irradiated with 30 μmol m −2 s −1 of blue light for indicated time. f Quantitative analysis of CRY2 degradation from immunoblots shown in ( e ). Data are presented as mean ± SD ( n = 3 individual immunoblots). CRY2 (B/D) = [CRY2/HSP90] blue / [CRY2/HSP90] dark . The best fitted curves with one phase decay of nonlinear regression were shown. CRY2 and HSP90 were detected with anti-CRY2 antibody and anti-HSP90 antibody, respectively. HSP90 is used as a loading control. Arrows indicate phosphorylated CRY2. The above experiments were repeated at least three times with similar results. Full size image LRBs interact with photoexcited and phosphorylated CRY2 Given that a substrate receptor of E3 ubiquitin ligases must physically interact with the substrate, we examined the CRY2/LRB interaction (Fig. 3 ), using the co-immunoprecipitation (co-IP) assays of proteins co-expressed in the heterologous HEK293T (Human Embryo Kidney 293T) cells as we previously reported [14] . Because we have previously shown that the blue light-induced phosphorylation of CRY2 is required for CRY2 ubiquitination and degradation, and that PPK1 is one of the four related protein kinases that specifically phosphorylate photoexcited CRY2 [18] , [20] , we tested CRY2/LRB interaction in the presence of the wild-type PPK1 in response to blue light in HEK293T cells. Results of this experiment show that LRB1 and LRB2 preferentially interact with phosphorylated CRY2 in HEK293T cells co-expressing PPK1, but only when cells were exposed to blue light (Fig. 3a, b ). LRB2 failed to interact with the photo-insensitive CRY2 D387A mutant that does not bind the FAD (Flavin Adenine Dinucleotide) chromophore [36] (Fig. 3c ), which is consistent with the light dependence of CRY2/LRB interaction. LRB2 failed to interact with CRY2 in light-treated HEK293T cells co-expressing the catalytically inactive PPK1 D267N (Fig. 3d ), which is consistent with the phosphorylation dependence of CRY2/LRB interaction. These results support a hypothesis that LRBs directly and specifically interact with photoexcited and phosphorylated CRY2. Fig. 3: LRBs interact with phosphorylated CRY2 in the HEK293T cells. a Co-immunoprecipitation (co-IP) assays showing the blue light and phosphorylation-dependent interaction of LRB1 and CRY2 in heterologous HEK293T cells. Immunoprecipitations (IP) were performed with Flag-conjugated beads. The IP (LRB1) and co-IP (CRY2) products were detected with anti-Flag and anti-CRY2 antibodies, respectively. PPK1 was detected with anti-HA antibody. b Co-IP assays showing the blue light and phosphorylation-dependent interaction of LRB2 and CRY2 in HEK293T cells. The experiments were performed as in ( a ). c Co-IP assays showing that LRB2 failed to interact with the photo-insensitive CRY2 D387A mutant. The experiments were performed as in ( a ), except that the IP (CRY2 and CRY2 D387A ) and co-IP (LRB2) products were detected with anti-CRY2 and anti-Myc antibodies, respectively. d Co-IP assays showing the phosphorylation-dependent interaction of LRB2 and CRY2 interaction in HEK293T cells. The experiments were performed as in ( a ). PPK1 D267N , catalytically inactive PPK1. e – f Co-IP assays showing the interaction between CRY2 CCE domain and LRB2. IP was performed with Flag-conjugated beads. The IP (PHR2 and CCE2) and co-IP (LRB2) products were detected with anti-Flag and anti-Myc antibodies, respectively. PHR2, photolyase homologous region of CRY2; CCE2, CRY2 C-terminal extension. The cells were treated with blue light (+ Blue; 100 μmol m −2 s −1 ) for 2 h or kept in the dark (-Blue). Arrows show phosphorylated CRY2. The above experiments were repeated three times with similar results. Full size image We next examined the CRY2/LRB interaction in plant cells, using the BiFC (Bimolecular Fluorescence Complementation) assay in Arabidopsis leaves [37] (Fig. 4a ) and split-luciferase assay in tobacco ( Nicotiana benthamiana ) leaves (Fig. 4b, c ). Results of the BiFC assay show strong BiFC signals between CRY2 and LRB1 or CRY2 and LRB2 (Fig. 4a ). In contrast, no BiFC signal was detected between the photo-insensitive CRY2 D387A and LRB1 or CRY2 D387A and LRB2 (Fig. 4a ). These results clearly demonstrate the direct interaction of CRY2 and LRB proteins in vivo. Consistently, the split-luciferase assays suggest the direct interaction between CRY2 and LRBs that contains deletion of the BTB domain (Fig. 4b, c ). Given the common affinity of BTB to Cullin 3 (Cul3) [31] , [38] , this experiment argues that the CRY2/LRB interaction is independent from BTB domain of LRBs or LRB/Cullin interaction. CRY2/LRB complexes are also detected by the co-IP (co-immunoprecipitation) assays in transgenic Arabidopsis seedlings stably co-expressing Flag-GFP-tagged CRY2 (FGFP-CRY2) and Myc-LRB1 or FGFP-CRY2 and Myc-LRB2 (Fig. 4d, e ). The co-IP assays detected increasing amount of the CRY2/LRB complexes in etiolated seedlings exposed to blue light or in seedlings grown in LD and continuous white light (Fig. 4d, e ). These results support a hypothesis that LRBs complex with CRY2 in a light-dependent manner and that LRBs act as the substrate receptors of Cul3 LRBs for the blue light-dependent CRY2 ubiquitination. It is noticed that the extent of photo-promotion of the accumulation of CRY2/LRB complexes in Arabidopsis seedlings is not as strong as that detected in light-treated heterologous HEK293T cells in the presence of PPK1 (Fig. 3 ) or that of blue light-induced CRY2 homooligomerization detected in Arabidopsis (Fig. 4d, e ). These results are consistent with the notions that CRY2 oligomerization is the primary photoreaction of the CRY2 photoreceptor and that LRBs interact with CRY2 to facilitate CRY2 degradation in vivo, but not in heterologous HEK293T cells. Fig. 4: LRBs interact with CRY2 in vivo. a Confocal microscopic images showing BiFC signals of indicated protein pairs transiently expressed in Arabidopsis leaves. The Hoechst 33342 (which is used to stain the nuclei) and GFP (BiFC) signals are shown. The relative intensity of CRY2/LRB interaction was presented as BiFC ratio, calculated as BiFC ratio = [GFP intensity] nuclei / [Hoechst 33342 intensity] nuclei . BiFC ratio (mean ± SD), total number of quantified images and nuclei are shown blow the images. CRY2 D387A , photo-insensitive CRY2, is used as the negative control. Scale bars, 10 μm. b Split-luciferase complementation assays showing the interactions of LRB1 and CRY2 or LRB2 and CRY2 in tobacco. Indicated split-LUC protein pairs were transiently co-expressed in N. benthamiana with FGFP-PPK1. LRB1ΔBTB, LRB1 with deletion of BTB domain (143-212 aa); LRB2ΔBTB, LRB2 with deletion of BTB domain (145-250 aa). c Quantification of split-luciferase complementation assays shown in ( b ). Data was shown as mean ± SD ( n = 3 individual experiments). d – e Co-immunoprecipitation assays showing the interactions of LRB1 and CRY2 ( d ) or LRB2 and CRY2 ( e ) in Arabidopsis . 7-day-old seedlings expressing Myc-LRB or co-expressing FGFP-CRY2 and Myc-LRB were grown in the dark and then treated with blue light (100 μmol m −2 s −1 ) for the indicated time, or grown in long days (LD, 16 h light/ 8 h dark) and continuous white light (cWL). Plant extracts were immunoprecipitated by GFP-trap beads. The IP and co-IP products were detected with anti-Flag and anti-Myc antibodies, respectively. Co-IP experiments of 7-day-old seedlings co-expressing FGFP-CRY2 and Myc-CRY2 were performed in parallel as positive controls. The relative interaction intensity of CRY2/LRB or CRY2/CRY2 is calculated by [Co-IP intensity] / [IP intensity] and shown blow the immunoblots. The above experiments were repeated twice with similar results. Full size image LRBs and COP1 are required for the photoresponsive polyubiquitination of CRY2 To test whether the Cul3 LRBs and Cul4 COP1/SPAs E3 ubiquitin ligases catalyze blue light-dependent CRY2 ubiquitination, we performed three independent experiments. In the first two experiments, we prepared transgenic plants overexpressing FGFP-CRY2 in the wild-type (WT), the strong ( lrb1lrb2-1lrb3 ) or weak ( lrb1lrb2-2lrb3) alleles of the lrb123 triple mutant (Fig. 5a, b, d ), and the cop1 mutant backgrounds (Fig. 5c, d ). In the third experiment, we prepared double-tagged transgenic lines that overexpress FGFP-CRY2 with either the Myc-tagged LRB (Myc-LRB1, Myc-LRB2) or the Myc-tagged COP1 (Myc-COP1) (Fig. 5e ). In the first experiment, polyubiquitinated proteins were indiscriminately precipitated using the TUBE2 (Tandem Ubiquitin Binding Entity 2)-conjugated beads [39] , and the TUBE2-enriched proteins were analyzed by immunoblots probed with the anti-ubiquitin or anti-CRY2 antibodies (Fig. 5a–c ). This experiment detected a high level of polyubiquitination of CRY2 in blue light-treated wild-type background seedlings (Fig. 5a–c ). However, little ubiquitinated CRY2 was detected in etiolated seedlings or in blue light-treated lrb123 or cop1 mutant background seedlings (Fig. 5a–c ). In the other two experiments, FGFP-CRY2 were immunoprecipitated by the GFP-trap beads, and the level of polyubiquitination of FGFP-CRY2 was analyzed by immunoblots probed against anti-ubiquitin antibody (Fig. 5d, e ). In etiolated seedlings exposed to blue light, a high level of ubiquitinated FGFP-CRY2 was detected in the wild-type seedlings overexpressing FGFP-CRY2. In contrast, a lower level of ubiquitinated FGFP-CRY2 was detected in lrb1lrb2-2lrb3 weak allele, whereas almost no ubiquitinated FGFP-CRY2 was detected in the lrb1lrb2-1lrb3 strong allele or the cop1 mutant seedlings transgenically overexpressing FGFP-CRY2 (Fig. 5d ). In comparison to FGFP-CRY2 overexpressed in the wild-type background, the blue light-induced polyubiquitination of FGFP-CRY2 is enhanced in plants co-overexpressing LRB1, LRB2, or COP1 (Fig. 5e ). Longer exposures of the chemiluminescence (Fig. 5d , bottom) demonstrate residual polyubiquitinations of CRY2 in either lrb123 or cop1 mutant and partial functional redundancy of the two E3 ligases. The minor ubiquitination signals detected in etiolated seedlings may result from basal activities of the enzymes or background signals. Taken together, results of those three independent experiments all support the hypothesis that two distinct E3 ubiquitin ligases, Cul3 LRBs and Cul4 COP1/SPAs , can both catalyze blue light-dependent polyubiquitination of CRY2 in vivo. Fig. 5: LRBs and COP1 are both required for CRY2 ubiquitination. Immunoblots showing the ubiquitination of FGFP-CRY2 in indicated genotypes. 7-day-old etiolated seedlings constitutively expressing FGFP-CRY2 in indicated genotypes were pretreated with MG132 and kept in the dark or exposed to 30 μmol m −2 s −1 of blue light for 5, 10, and 15 min. The blue light treated samples (5, 10, and 15 min) were pooled together while performing immunoprecipitation for ( a – e ). a – c Total ubiquitinated proteins were purified by TUBE2-conjugated beads. Immunoprecipitated proteins were analyzed by immunoblots probed with anti-ubiquitin antibody (α-Ubq) or anti-CRY2 antibody (α-CRY2). The extent of CRY2 ubiquitination was shown below the immunoblots, calculated as [CRY2-Ubq intensity] IP /[Ubq intensity] IP . d – e FGFP-CRY2 proteins were purified with GFP-trap beads. Immunoprecipitated proteins were analyzed by immunoblots probed with anti-ubiquitin antibody (α-Ubq), anti-Flag antibody (α-Flag) or anti-Myc antibody (α-Myc) for detecting epitope-tagged proteins. The extent of CRY2 ubiquitination is calculated as [CRY2-Ubq intensity] IP /[Flag intensity] IP with the short exposure immunoblots and shown below the immunoblots. S. exp or L. exp: short or long chemiluminescence exposures of immunoblots. D, dark treatment; B, blue light treatment. The above experiments were repeated at least twice with similar results. Full size image COP1 and LRBs interact with different structural elements of CRY2 We wish to understand different mechanisms governing the activities of COP1 and LRBs with respect to CRY2 ubiquitination. Most presently known light-dependent CRY2-interacting proteins interact with the photon-sensing PHR domain of CRY2 [3] . However, COP1 is one of the few exceptions. COP1 binds to the CCE domain of CRYs regardless of light in vitro or in yeast cells [33] , [34] , [35] , although COP1 binds to CRY2 in the light-dependent manner in vivo [40] , [41] . Like COP1, LRB2 also interacts with the CCE domain of CRY2 in heterologous HEK293T cells (Fig. 3e, f ). However, in contrast to COP1 that interacts with CRYs regardless of light in vitro or in yeast cells, LRBs preferentially interact with phosphorylated CRY2 in the blue light-dependent manner in HEK293T cells (Fig. 3a–d ). Given that analyses of molecular interactions of plant proteins in heterologous yeast cells, HEK293T cells, or in vitro are essentially equivalent, we reasoned that CRY2 may interact with COP1 or LRBs via different structural elements and/or respond to the photoresponsive CRY2 conformation changes differently. We investigated this question by analyses of the CRY2 P532L mutation that is impaired at the VP motif (Fig. 6a ). The VP motif is a conserved COP1-binding motif of many substrates of the Cul4 COP1/SPAs E3 ligase, including CRY2 [42] , [43] . We previously reported that the CRY2 P532L mutation impaired at the VP motif (Fig. 6a ) loses all the physiological activities tested but retains many photochemical properties of CRY2, including blue light-induced oligomerization, phosphorylation, ubiquitination, and degradation [15] . We first compared the relative activity of FGFP-CRY2 and FGFP-CRY2 P532L , using the hypocotyl inhibition assay in transgenic plants expressing the respective recombinant protein at similar levels in the cry1cry2 mutant background (Supplementary Fig. 3a ). Transgenic seedlings expressing FGFP-CRY2 P532L showed no obvious activity mediating light inhibition of hypocotyl elongation under all light intensities of blue light tested (Fig. 6b , Supplementary Fig. 3b ). This result confirmed our previous report that CRY2 P532L is a loss-of-function mutation [15] . We then compared the kinetics of blue light-induced degradation of FGFP-CRY2 and FGFP-CRY2 P532L , using the same transgenic lines (Fig. 6c, d ). In transgenic seedlings, the mutant recombinant protein FGFP-CRY2 P532L is degraded in response to blue light as we previously reported [15] , although it appears to degrade slower than its wild-type counterpart (Fig. 6c, d ). The apparent half-life of FGFP-CRY2 P532L is more than twice that of FGFP-CRY2 (Fig. 6d ). When co-expressed with PPK1 in HEK293T cells, both the wild-type CRY2 and the CRY2 P532L mutant protein exhibits clear blue light-dependent phosphorylation (Fig. 6e, f ). In HEK293T cells co-expressing SPA1, COP1 interacts with CRY2 in the light-dependent manner with both phosphorylated and unphosphorylated CRY2, whereas neither the photo-insensitive CRY2 D387A mutant nor the COP1-insensitive CRY2 P532L mutant interact with COP1 or SPA1 (Fig. 6e ). LRB2 preferentially interacts with photoexcited and phosphorylated CRY2, as well as the photoexcited and phosphorylated CRY2 P532L mutant to the similar extent (Fig. 6f ). These results are consistent with that CRY2 P532L remains photoresponsive in vivo [15] and that CRY2 P532L undergoes blue light-dependent ubiquitination and degradation in vivo (Fig. 6c, d ). Since the CRY2 P532L mutant does not interact with COP1, these results confirm that COP1 and LRB2 interact with different structural elements of CRY2. Taken together, results of our analyses of the CRY2 P532L mutant further supports the hypothesis that Cul3 LRBs is the second type of E3 ligase required for blue light-dependent CRY2 ubiquitination and degradation. Fig. 6: LRBs and COP1 interact with different structural elements of CRY2. a A schematic diagram depicting the CRY2 P532L mutation. PHR, photolyase homologous region; CCE, CRY C-terminal extension; DQQVPSAV, VP motif in CRY2; numbers, amino acid positions. b Hypocotyl length of 6-day-old seedlings of indicated genotypes grown under blue light of different light intensities. Data were shown as mean ± SD. c Immunoblots showing degradation of FGFP-CRY2 or FGFP-CRY2 P532L in 7-day-old etiolated seedlings irradiated with blue light (100 μmol m −2 s −1 ) for the indicated time. Immunoblots were probed with anti-CRY2 and anti-HSP90 antibodies. d Quantitative analysis of CRY2 degradation from immunoblots shown in ( c ), n = 3 individual immunoblots. The best fitted curves with one phase decay of nonlinear regression were shown. CRY2 (B/D) = [CRY2/HSP90] blue / [CRY2/HSP90] dark . T 1/2 indicates the time required for 50% degradation. e – f Co-IP assays showing the lack of CRY2 P532L /COP1 interaction ( e ) and the blue light- and phosphorylation-dependent CRY2 P532L /LRB2 interaction ( f ) in HEK293T cells. Transfected cells were either kept in the dark (− Blue) or treated with 100 μmol m −2 s −1 blue light for 2 h (+ Blue). CRY2 D387A is used as a negative control. Anti-Flag, anti-Myc or anti-HA antibodies were used for detecting indicated tagged proteins. Arrows indicate phosphorylated CRY2. g Co-IP results showing the photooligomerization of CRY2 P532L in HEK293T cells. Transfected cells were irradiated with blue light (30 μmol m −2 s −1 ) for indicated time. CRY2 P532L tagged with Flag or Myc were detected with anti-Flag and anti-Myc antibodies, respectively. h Comparison of photooligomerization kinetics of CRY2 and CRY2 P532L in HEK293T cells. Co-IP (α-Myc) signals was normalized to the corresponding IP (α-Flag) signals, and the dark oligomerization level was set as 1. O 50 indicates the time required to reach 50% saturation of CRY2 photooligomerization. The best fitted curves with one phase association of nonlinear regression were shown. i Co-IP results showing the dark reversion of CRY2 P532L photooligomers in HEK293T cells. The cells were treated with 30 μmol m −2 s −1 blue light for 5 min then moved to the darkness for indicated time. j Comparison of the dark reversion dynamics of CRY2 and CRY2 P532L photooligomers in HEK293T cells. Similar analyses were performed as in ( h ), except that the oligomerization level in blue was set as 1. T 1/2 indicates the time required to reverse 50% of CRY2 photooligomers into monomers. The best fitted curves analyzed with one phase decay of nonlinear regression were shown. CRY2 photooligomerization and dark reversion data shown in ( h ) and ( j ) were extracted from the published paper [15] with permission. The above experiments were repeated at least twice with similar results. Full size image The notion that Cul3 LRBs and Cul4 COP1/SPAs regulate CRY2 predominantly in the early or prolonged state of light exposure, respectively, seems inconsistent with the kinetics of CRY2 P532L degradation in vivo (Fig. 6c, d ). Because the CRY2 P532L interacts with LRB2 but not COP1 (Fig. 6e, f ), its degradation is expected to mimic that of the wild-type CRY2 in the cop1 mutant (Fig. 2 ). Instead, the kinetics of CRY2 P532L degradation is more like that of the wild-type CRY2 in the lrb123 triple mutant (Fig. 2 ). This seemingly perplexing phenomenon may be explained by the unusual photochemical characteristics of the CRY2 P532L mutant. Photoexcited CRY2 P532L monomers exhibit increased affinity among themselves in comparison to the wild-type CRY2 (Fig. 6g, h ) without obvious change of the rate or affinity in the dark-reversion reaction (Fig. 6i, j ). Because photooligomerization is necessary for all light-dependent reactions of CRY2, including photoresponsive ubiquitination and degradation [14] , [15] , it is conceivable that the unusual photochemical characteristics of the CRY2 P532L mutant may change its relationship with various regulators in vivo, including LRBs or 26S proteosomes, to alter its degradation kinetics in the unexpected manner. Taken together, the results of our experiments argue that two types of substrate receptors, COP1 and LRBs, interact with CRY2 via distinct structural elements of CRY2 to enable the blue light-induced CRY2 ubiquitination and degradation by the respective E3 ubiquitin ligases, Cul3 LRBs and Cul4 COP1/SPAs . In this study, we demonstrate that, in addition to Cul4 COP1/SPAs , the E3 ubiquitin ligases Cul3 LRBs is required for blue light regulation and function of CRY2 (Fig. 7a ). Cul3 LRBs appears capable of targeting photoexcited and phosphorylated CRY2 for a rapid ubiquitination and degradation, whereas Cul4 COP1/SPAs is responsible for the sustained ubiquitination and degradation of CRY2 in plants under prolonged light exposure. The differential regulation of CRY2 turnover in response to different light conditions appears necessary for the optimal photoresponses of plants grown in nature. LRBs and COP1 interact with different structural elements of CRY2, which explain, at least partially, the different kinetic features of the LRB- and COP1-dependent CRY2 degradation in response to blue light. Photoresponsive expression of LRBs may also play a role in the light regulation of CRY2 turnover. Blue light positively regulates LRB1 and LRB2 protein expression (Fig. 7b–e ). The abundance of recombinant LRB proteins in transgenic plants expressing LRB1 or LRB2 driven by either the respective native promoters or the ACT2 constitutive promoter increase in response to blue light. Because Cul4 COP1/SPAs -dependent ubiquitination and 26S proteosome pathway is best known for degradation of photo-signaling proteins in darkness, it is tempting to speculate that Cul4 COP1/SPAs may play a role in the regulation of the LRB proteins expression, and the CRY2-mediated light inhibition of Cul4 COP1/SPAs may lead to increased LRB protein accumulation, accelerated turnover of not only photoexcited CRY2 but also photoexcited phyB, and sustained overall photosensitivity of plants grown in nature (Fig. 7a ). However, this hypothesis remains to be tested directly. Fig. 7: Blue light positively regulates LRBs protein abundance in plants. a A hypothetic model depicting the degradation of CRY2 by LRBs and COP1 E3 ubiquitin ligases. CRY2 exists as inactive monomers in darkness (grey). Upon blue light exposure, CRY2 undergoes photoexcitation, oligomerization, and phosphorylation to become photoactive. Photoactivated CRY2 then were targeted by two distinct E3 ubiquitin ligases, LRBs, and COP1, for degradation. Minus sign in a circle, indicates negative charge; dashed line, indicates a hypothetical mechanism. b – e Representative immunoblots (top) and a quantitative analysis (bottom) showing the expression of recombinant LRB proteins in transgenic plants driven by native promoters ( b , d ) or the ACT2 constitutive promoter ( c , e ). Seedlings were grown in darkness or continuous blue light (50 μmol m −2 s −1 ) for 5, 6, or 7 days. Proteins were extracted and subjected to western blot analysis. LRBs and HSP90 were detected with anti-Flag and anti-HSP90 antibodies, respectively. HSP90 is used as a loading control. Data were shown as mean ± SD ( n = 3 individual immunoblots). The above experiments were repeated at least three times with similar results. Full size image LRBs and COP1 apparently interact with CRY2 differently: LRBs interacts with photoexcited and phosphorylated CRY2, whereas COP1 interacts with CRY2 regardless of its phosphorylation states. This result would be consistent with CRY2 interacting with COP1 or LRBs via different structural elements. Photoexcitation of CRYs may result in different conformational changes and interactions with different proteins. First, photoexcited CRYs may undergo initial conformational change associated with CRY oligomerization, which have been directly shown by several recent structural studies of the PHR domain of CRY2 [3] , [16] , [17] , [44] . Second, light-induced phosphorylation of CRYs may result in electrostatic repelling of the PHR and CCE domains of CRYs and open conformation of CRYs, which has been deduced from the conventional structure-function studies [35] , [45] . However, technical difficulties, including the intrinsically disordered nature of the CCE domain of CRY2, has prevented a direct test of conformational changes of the CRY2 holoprotein. Because COP1 interacts with CRY2 regardless of CRY2 phosphorylation, whereas LRBs primarily interacts with phosphorylated CRY2 (Fig. 3 , Fig. 6e, f ), we propose that the first type of conformational change is primarily responsible for the photoresponsive interaction of COP1 and CRY2, whereas the second type of conformational change of CRY2 is primarily responsible for the photoresponsive interaction of LRBs and CRY2. These hypotheses, however, remain to be further tested. It is interesting that plants evolved with two distinct E3 ubiquitin ligases to regulate a CRY photoreceptor by different modes of interaction under different light conditions. In mammals, two related Cul1-based E3 ligases, SCF FBXL3 and SCF FBXL21 , act to promote ubiquitination and degradation of CRYs in the nucleus and cytoplasm, respectively, to control the period of the circadian clock [8] . In Drosophila, Jetlag of a Cul1-based E3 ligase and Brwd3 of a Cul4-based E3 ligase regulate ubiquitination and degradation of dCRY-dependent circadian rhythm [9] , [10] . Cul4 Brwd3 mediates light-dependent ubiquitination and degradation of dCRY, whereas Cul1 Jetlag interacts with dCRY to catalyze ubiquitination of the dCRY-interacting protein TIM [10] , [46] . Decreased TIM may enhance interaction of dCRY with its E3 ligases to accelerate its degradation in light. These studies demonstrate that multiple E3 ligases are needed to regulate the activity of a CRY to control the circadian clock. The results of this study argue that plant CRY2 is also controlled by two distinct E3 ligases, and that the delicate control of the abundance of CRYs is evolutionarily conserved for not only circadian rhythms in animals but also photomorphogenesis in plants. Our finding that Cul3 LRBs or Cul4 COP1/SPAs catalyze CRY2 ubiquitination in different light conditions, to promote rapid or prolonged degradation of CRY2, respectively, highlights the importance of photoreceptor turnover in the regulation of photosensitivity of plants. Altogether, these results appear to argue for the similar selection pressure to maintain multiple mechanisms regulating the abundance of CRY proteins during evolution of both animal and plant lineages. The complex mechanism regulating CRY2 turnover is likely evolved to optimize photomorphogenesis under natural light conditions. In this regard, it is particularly interesting that Cul3 LRBs has been previously shown to be the E3 ligase of PIF3 and critical for the function of phyB and phytochrome-dependent photoresponses [30] , [31] . Our finding that Cul3 LRBs also catalyzes blue light-dependent ubiquitination of CRY2 to regulate blue light-dependent photomorphogenesis argues for a previously unrecognized mechanism toward a better understanding of how plants respond to light in the nature white light conditions. Plasmid construction All plasmids used in this study were generated by In-Fusion Cloning methods ( https://www.takarabio.com/products/cloning/in-fusion-cloning ). The sequences subcloned into plasmids were verified by Sanger sequencing. The mammalian cell expression vectors used in this study were made with pQCMV-Flag-GFP (Supplementary Fig. 4 ), pQCMV-GFP (Supplementary Fig. 4 ), and pCMV-Myc [20] . pQCMV-Flag-GFP vector was modified from the commercial plasmid pEGFP-N1 (Clontech), which allows the inserted gene expressed under control of the CMV promoter and fused with dual in-frame tags of Flag and GFP. pQCMV-GFP vector was further modified from pQCMV-Flag-GFP by removing the coding sequence of Flag tag. pCMV-Myc vector was described previously [20] . To generate plasmids expressing Flag-LRB1, Flag-LRB2, Flag-CRY2, and Flag-CRY2 D387A , the coding sequences (CDS) of all the above genes were amplified either from Arabidopsis cDNA or plasmids made before by PCR, the purified PCR products were then subcloned into SpeI/KpnI-digested pQCMV-Flag-GFP vector through in-fusion. Myc-LRB1 , Myc-LRB2 , Myc-CRY2 , Myc-SPA1, and Myc-COP1 plasmids were prepared by cloning the CDS of the genes into the BamHI site of pCMV-Myc vector. For plasmids expressing HA-PPK1 and HA-PPK1 D267N , the coding sequences of PPK1 and PPK1 D267N were PCR-amplified from plasmids made before by using the primers, of which a 2x HA coding sequence was attached to the 5’ end of forward primer, and introduced into SpeI/KpnI-digested pQCMV-GFP vector by in-fusion. 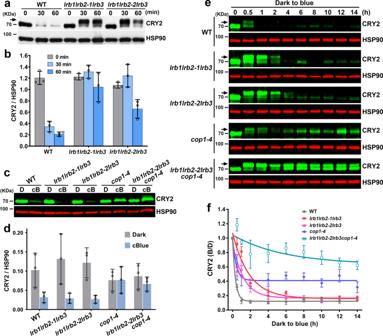Fig. 2: LRBs and COP1 regulate the rapid or prolonged proteolysis of CRY2, respectively. aRepresentative immunoblots showing the abundance of endogenous CRY2 in the 7-day-old etiolated wild type (WT) andlrb123mutants irradiated with 30 μmol m−2s−1of blue light for the indicated time.bQuantitative analysis of CRY2 abundance from immunoblots shown in (a). Data are presented as mean ± SD (n= 3 individual immunoblots).cRepresentative immunoblots showing the abundance of endogenous CRY2 in seedlings of indicated genotypes grown in darkness (D) or continuous blue light (cB, 30 μmol m−2s−1).dQuantitative analysis of CRY2 abundance from immunoblots shown in (c). Data are presented as mean ± SD (n= 3 individual immunoblots).eRepresentative immunoblots showing degradation of the endogenous CRY2 in 7-day-old etiolated seedlings irradiated with 30 μmol m−2s−1of blue light for indicated time.fQuantitative analysis of CRY2 degradation from immunoblots shown in (e). Data are presented as mean ± SD (n= 3 individual immunoblots). CRY2 (B/D) = [CRY2/HSP90]blue/ [CRY2/HSP90]dark. The best fitted curves with one phase decay of nonlinear regression were shown. CRY2 and HSP90 were detected with anti-CRY2 antibody and anti-HSP90 antibody, respectively. HSP90 is used as a loading control. Arrows indicate phosphorylated CRY2. The above experiments were repeated at least three times with similar results. The gene-specific primers for constructs used for expressing recombinant proteins in HEK293T cells are listed in Supplementary Table 2 . The BiFC constructs were built with the vectors described previously [47] . The coding sequences of LRB1 (AT2G46260), LRB2 (AT3G61600), CRY2 (AT1G04400), and CRY2 D387A were PCR-amplified and cloned into pDONR/Zeo entry vector through BP reaction (Gateway™ BP Clonase™ II Enzyme mix, Cat. # 11789020, Invitrogen). The entry constructs were then introduced into the destination vector pX-nYFP (N-terminus of YFP fused to C-terminus of genes) or pcCFP-X (C-terminus of CFP fused to N-terminus of genes) by LR reaction (Gateway™ LR Clonase™ II Enzyme mix, Cat. # 11791020, Invitrogen). The gene-specific primers of Gateway cloning for constructs used for BiFC assys are listed in Supplementary Table 2 . The split-LUC constructs were made with the vectors described previously [48] . CRY2 were fused to the C-terminus of cLUC (the C-terminus of Luciferase). LRB1ΔBTB were generated by seamlessly connecting two fragments, 1-426 bp and 637-1683 bp of LRB1 coding sequence, with 15 bp overlaps, by infusion cloning method. LRB2ΔBTB were generated with two fragments, 1-432 bp and 751-1683 bp of LRB2 coding sequence through the same method as making LRB1ΔBTB . LRB1ΔBTB and LRB2ΔBTB were then fused to the N-terminus of nLUC (the N-terminus of Luciferase) by in-fusion. The primers for constructs used for Split-LUC assays are listed in Supplementary Table 2 . pFGFP (Supplementary Fig. 5 ) and pDT1H (Supplementary Fig. 5 ) binary vectors were used for creating overexpression transgenic lines. The pFGFP binary vector was modified from pCambia3301 [20] , which allows the interested genes to express under Actin2 promoter and fuse with 2x Flag and GFP tags. The pDT1H binary vector, possessing two independent expression cassettes that allows two genes to assemble into one vector, was modified from previously published vector pDT1 [49] by replacing the BAR gene with HPT gene to convert basta resistance to hygromycin resistance in plants. The CDS of LRB1 , LRB2 , CRY2, and CRY2 P532L were cloned into BamHI-digested pFGFP vector to generate FGFP-LRB1 , FGFP-LRB2 , FGFP-CRY2 , FGFP-CRY2 P532L with 2x Flag and GFP tags fused to N-terminus of the genes. The native promoters of LRB1 and LRB2 were cloned into SacI/SpeI-digested FGFP-LRB1 and FGFP-LRB2 to generate ProLRB1::FGFP-LRB1 and ProLRB2::FGFP-LRB2 , respectively. The CDS regions of LRB1 , LRB2, and COP1 (AT2G32950) were cloned into the BamHI site of pDT1H vector to produce Myc-LRB1 , Myc-LRB2, and Myc-COP1 with 4x Myc tags fused to N-terminus of the genes. The primers for constructs used for plant transformation are listed in Supplementary Table 2 . Plant materials and growth conditions All mutants used in this study are in the Arabidopsis thaliana Columbia ecotype background. The cry1cry2 double mutant were described as previously [32] . The lrb1lrb2-1lrb3 ( lrb1 , Salk_145146; lrb2-1 , Salk_001013; lrb3 , Salk_082868) and lrb1lrb2-2lrb3 ( lrb2-2 , Salk_044446) triple mutants were gifts from Dr. Peter Quail and as described previously [30] , [31] . cop1-4 and cop1-6 are weak mutant alleles of COP1 as previously described [50] . cry1cry2lrb1lrb2-2lrb3 and lrb1lrb2-2lrb3cop1-4 mutants were generated by crossing. The genotypes of lrb123 mutants were verified by PCR using the primers listed in Supplementary Table 2 . cop1-4 mutant was verified by PCR using the primers listed in Supplementary Table 2 , followed by Sanger sequencing to confirm the point mutation of COP1 gene. cry1cry2 mutant was verified by western blots using antibodies against CRY1 and CRY2 proteins. All transgenic lines were generated via Agrobacterium tumefaciens –mediated floral-dip method [51] . The wild-type plants used for transformation in this study are rdr6-11 , which suppresses gene silencing [52] . For in vivo ubiquitination study, FGFP-CRY2 was introduced into rdr6-11 , lrb1lrb2-1lrb3 , lrb1lrb2-2lrb3 , cop1-4 and cop1-6 background. The FGFP-CRY2/Myc-LRB1 double-overexpression lines were prepared by introducing FGFP-CRY2 into Myc-LRB1/rdr6-11 plants. The transgenic T1 populations were screened on MS plates containing 25 mg/L Glufosinate-ammonium (cat # CP6420, Bomei Biotechnology) and 25 mg/L hygromycin (cat # 10843555001, Roche), and western blots were performed to confirm the expression of both proteins. The same method was used for generating FGFP-CRY2/Myc-LRB2 and FGFP-CRY2/Myc-COP1 double-overexpression lines. For experiments comparing the hypocotyl phenotype and protein degradation kinetics of FGFP-CRY2 and FGFP-CRY2 P532L , FGFP-CRY2 and FGFP-CRY2 P532L were introduced into cry1cry2rdr6 background. The cry1cry2rdr6 were generated by crossing cry1-304 [32] , cry2-1 [12] , and rdr6-11 [52] . The transgenic lines were screened on MS plates with 25 mg/L Glufosinate-ammonium, and lines with similar protein expression level of FGFP-CRY2 and FGFP-CRY2 P532L were used for analysis. For lrb123 mutant blue-light hypersensitivity phenotype rescue experiments, FGFP-LRB2 and Myc-LRB2 were transformed into lrb1lrb2-2lrb3 background. For routine maintenance, Arabidopsis thaliana were grown under long day conditions (16 h light / 8 h dark) at 22 °C. For hypocotyl phenotype analysis, seedlings were grown on MS plates with 3% sucrose at 20–22 °C for 6 days under different light conditions. Light-emitting diode (LED) was used to obtain monochromatic light (blue light, peak 465 nm, half-bandwidth of 25 nm; red light, peak 660 nm, half-bandwidth of 20 nm; far-red light, peak 735 nm, half-bandwidth of 21 nm). For endogenous CRY2 degradation analysis in WT, lrb123 , cop1 and lrb123cop1 mutants, seedlings were grown in darkness on MS plates with 3% sucrose for 7 days, then subjected to 30 μmol m −2 s −1 blue light for the indicated time. For FGFP-CRY2 and FGFP-CRY2 P532L degradation analysis, seedlings were grown in darkness on MS plates with 3% sucrose for 7 days, then subjected to 100 μmol m −2 s −1 blue light for the indicated time. For immunoprecipitation of polyubiquitinated proteins, 7-day-old etiolated seedlings grown on MS medium containing 3% sucrose were treated with 50 μM MG132 (Cat # S2619, Selleck) in liquid MS in the dark overnight with gentle shaking, and then moved to 30 μmol m −2 s −1 blue light for 5, 10, and 15 min before harvest. Blue-light-induced CRY2 degradation assays For endogenous CRY2 degradation analysis, seedlings were grown in the dark for 7 days and then treated with 30 μmol m −2 s −1 of blue light for indicated time. For FGFP-CRY2 and FGFP-CRY2 P532L degradation analysis, seedlings were treated with 100 μmol m −2 s −1 of blue light. Tissues were homogenized by TissueLyser (QIAGEN). Proteins were extracted in equal tissue volume of protein extraction buffer [120 mM Tris pH 6.8, 100 mM EDTA, 4% w/v SDS, 10% v/v beta-mercaptoethanol, 5% v/v Glycerol, 0.05% w/v Bromophenol blue] [53] , heated at 100 °C for 8 min, centrifuged at 16000 rcf for 10 min, and analyzed by western blot. Proteins were separated in 10% SDS-PAGE, and transferred to nitrocellulose membranes (Pall Life Sciences). For immunoblot signals detected by enhance conventional chemiluminescent (ECL) method, membranes were blocked with 5% non-fat milk in PBST for 1 h, blotted with anti-CRY2 primary antibody (1:3000, homemade, produced in rabbit [12] ) in PBST for 1.5 h, washed 8 min x 3 times with PBST, blotted with anti-Rabbit-HRP (1:10000, cat # 31460, ThermoFisher) secondary antibody in PBST for 1.5 h, washed 8 min x 3 times with PBST and then incubated with ECL solution for X-ray film development. The membranes were then stripped with stripping buffer [0.2 M Glycine, pH 2.5] and re-probed with anti-HSP82 (1:10000, cat # AbM51099-31-PU, Beijing Protein Innovation) primary antibody and anti-Mouse-HRP (1:10000, cat # 31430, ThermoFisher) secondary antibody. Anti-HSP82 antibody from Oryza sativ a can also recognize Arabidopsis HSP90 protein [54] . Three independent blots were performed in parallel for quantification analysis. The quantification of protein intensity of ECL immunoblots was performed by ImageJ. For immunoblot signals detected by Odyssey CLx Infrared Imaging System (Li-COR), membranes were blocked with 0.5% casein in PBS for 1 h, blotted with anti-CRY2 (1:3000) and anti-HSP82 (1:10000) mixed primary antibodies in PBST with 0.5% casein for 1.5 h, washed 8 min x 3 times with PBST, blotted with Donkey anti-rabbit 790 (1:15000, cat # A11374, ThermoFisher) and Donkey anti-mouse 680 (1:15000, cat # A10038, ThermoFisher) mixed secondary antibodies in PBST with 0.5% casein for 1.5 h, washed 8 min x 3 times with PBST and then signals were captured with Odyssey CLx by Image Studio Lite software. Three independent blots were performed in parallel for quantification analysis. Quantification of signals were processed with Image Studio Lite software. CRY2 degradation curves were indicated by CRY2 (B/D) ratio, calculated as CRY2 (B/D) = [CRY2/HSP90] blue / [CRY2/HSP90] dark , and analyzed with one phase decay of nonlinear regression. Protein expression and co-immunoprecipitation in HEK293T cells Human embryonic kidney (HEK) 293T cells were cultured in Dulbecco’s modified Eagle’s medium (DMEM) supplemented with 10% (v/v) FBS, 100 mg/L streptomycin and 100 IU penicillin, in humidified 5% (v/v) CO 2 air at 37 °C. Cells were seeded at a density of approximately 8 × 10 5 cells/6-cm plate and the transfection were carried out with a calcium phosphate precipitation protocol. Briefly, different combinations of plasmid DNA (2~5 μg / construct) were mixed with 30 µl 2.5 M CaCl 2 and ddH 2 O to a total volume of 300 µl, then 300 µl of 2x HeBS [250 mM NaCl, 10 mM KCl, 1.5 mM Na 2 HPO 4 , 12 mM Dextrose and 50 mM HEPES, adjust the pH of the final solution to 7.05] was added drop by drop with vortex, and kept at room temperature for 5 min before applying to cells. The media were aspirated from each plate, DNA mixtures were gently added into plates and the plates were rotated gently to allow the mixtures to coat the entire plate. 3 ml of fresh media containing 25 μM chloriquine (cat # C6628, Sigma) were added to each plate and the plates were kept in the CO 2 incubator overnight. The next day, the media were changed with 3 ml of fresh media without chloriquine. 36–48 h after transfection, the cells were subjected to blue light treatment for indicated time, washed twice with cold PBS buffer and then harvested in liquid nitrogen for co-immunoprecipitation. Cells transfected with different plasmid DNA were lysed in 800 μl 1% Brij buffer [1% Brij-35, 50 mM Tris-HCl pH 8.0, 150 mM NaCl, 1 mM EDTA,1x Protease inhibitor cocktail, and 1x phosphatase inhibitor PhosSTOP] with rotating at 4 °C for 20 min. Cell lysates were centrifuged at 16,000 rcf for 10 min at 4 °C, and the supernatants were incubated with 20 μl Anti-FLAG M2 affinity gel (Cat. # F2426, Sigma) at 4 °C for 2 h with rotation. Beads were washed with 1% Brij buffer for 5 times. Proteins were competed from the beads with 35 μl 3xFlag peptide solution [500 ng/μl in 1% Brij buffer] for 30 min at room temperature with mixing. Elution was transferred to a new tube, mixed with 4XSDS sample buffer, denatured at 100 °C for 4 min and subjected to western blot analysis. Western blots were performed as described above. Primary antibodies used here were anti-Flag (1:1500, cat # F1804, Sigma), anti-Myc (1:5000, cat # 05-724, Millipore), and anti-HA (1:5000, cat # 12013819001, Roche), and secondary antibodies used were anti-Mouse-HRP (1:10000, cat # 31430, ThermoFisher) and anti-Rabbit-HRP (1:10000, cat # 31460, ThermoFisher). Bimolecular fluorescence complementation (BiFC) assay BiFC assays in Arabidopsis plants were performed as previously described methods with minor modifications [37] . Briefly, Agrobacteria AGL0 transformed with BiFC plasmids were grown in LB medium with 40 μM Acetosyringone and 1% Glucose in 28 °C shaker overnight. Agrobacteria were centrifuged at 5000 rcf for 10 min, washed once with washing buffer [10 mM MgCl 2 , 100 μM Acetosyringone] and resuspended in infiltration buffer [1/4 MS pH 6.0, 1% sucrose, 100 μM Acetosyringone, and 0.01% Silwet L-77] to 0.5 of OD600. The agrobacteria were infiltrated into 3–4 weeks old Arabidopsis leaves with syringe. Each BiFC assay was performed with at least 3 independent plants with 2–3 leaves infiltrated for each. Plant leaves were dried before kept in the dark for 24 h, and then moved back to long day conditions (16 h light/8 h dark) to grow for 2 more days. The infiltrated leaf samples were analyzed under a Leica TCS SP8X confocal microscope. Hoechst 33342 was used for nuclei staining. The quantification of fluorescence intensity was performed by ImageJ. Briefly, the images of GFP and Hoechst 33342 channels from the same field were stacked first, then the regions of nuclei were selected on the image of Hoechst 33342 channel. The integrated intensity of the selected regions over the entire stack were measured. The BiFC ratio of the selected regions were calculated as [GFP intensity] nuclei / [Hoechst 33342 intensity] nuclei for each image. Four to nine images (~40–100 nuclei in total) for each BiFC assay were used for quantification and the BiFC ratios were presented as mean ± SD (standard deviation). Split-luciferase (Split-LUC) assay Split-LUC plasmids were transformed into Agrobacteria AGL0. Each Agrobacteria with respective plasmid was grown in LB medium with 40 μM Acetosyringone and 1% Glucose in 28 °C shaker overnight. Agrobacteria were centrifuged at 5000 rcf for 10 min, washed once with washing buffer [10 mM MgCl 2 , 100 μM Acetosyringone] and resuspended in infiltration buffer [1/4 MS pH 6.0, 1% sucrose, 100 μM Acetosyringone, and 0.01% Silwet L-77] to 0.5 of OD600. Agrobacteria with the nLUC- or cLUC-fusion proteins were mixed at a ratio of 1:1 and were infiltrated into N. benthamiana leaves with syringe. Each split-LUC assay was performed with at least 3 leaves. The bacteria culture remained on the surface of plant leaves were dried before the plants were kept in the dark for 24 h, and then moved back to long day conditions (16 h light/8 h dark) to grow for 2 more days. Before the analysis, 1 mM D-luciferin with 0.01% Triton X-100 were sprayed on the leaves, and the leaves were kept in the dark for 20 min before signal detecting with Tanon-5200. The quantification of luminescence intensity was performed by ImageJ. Immunoprecipitation of ubiquitinated proteins in Arabidopsis 7-day-old etiolated seedlings were treated with 50 μM MG132 in liquid MS in the dark overnight with gentle shaking, and then treated with 30 μmol m −2 s −1 blue light for 5, 10, and 15 min before harvest. For each immunoprecipitation assay, about 3 g of seedlings were used. Seedlings were ground in liquid nitrogen and homogenized in 1.5x tissue volume of IP buffer [50 mM Tris-HCl pH 7.5, 150 mM NaCl, 1 mM EDTA, 1% Triton X-100, 20 mM NaF, and 1x Protease inhibitor cocktail] at 4 °C for 20 min with mixing. Lysates were centrifuged at 16,000 rcf for 15 min at 4 °C. A total of 100 μl of supernatant were saved as inputs. For total ubiquitinated protein purification, the supernatant for each sample was incubated with 30 μl Agarose-TUBE2 beads (cat # UM402M, LifeSensors) for 2 h at 4 °C with rotating. Then, beads were pelleted and washed four times with ice-cold IP buffer (without inhibitors). 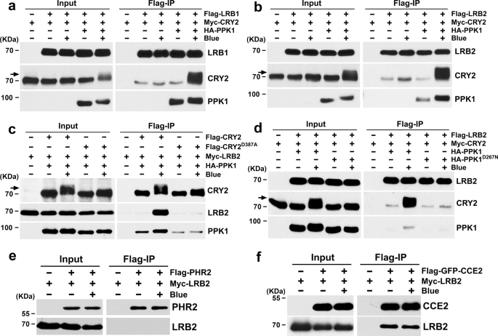Fig. 3: LRBs interact with phosphorylated CRY2 in the HEK293T cells. aCo-immunoprecipitation (co-IP) assays showing the blue light and phosphorylation-dependent interaction of LRB1 and CRY2 in heterologous HEK293T cells. Immunoprecipitations (IP) were performed with Flag-conjugated beads. The IP (LRB1) and co-IP (CRY2) products were detected with anti-Flag and anti-CRY2 antibodies, respectively. PPK1 was detected with anti-HA antibody.bCo-IP assays showing the blue light and phosphorylation-dependent interaction of LRB2 and CRY2 in HEK293T cells. The experiments were performed as in (a).cCo-IP assays showing that LRB2 failed to interact with the photo-insensitive CRY2D387Amutant. The experiments were performed as in (a), except that the IP (CRY2 and CRY2D387A) and co-IP (LRB2) products were detected with anti-CRY2 and anti-Myc antibodies, respectively.dCo-IP assays showing the phosphorylation-dependent interaction of LRB2 and CRY2 interaction in HEK293T cells. The experiments were performed as in (a). PPK1D267N, catalytically inactive PPK1.e–fCo-IP assays showing the interaction between CRY2 CCE domain and LRB2. IP was performed with Flag-conjugated beads. The IP (PHR2 and CCE2) and co-IP (LRB2) products were detected with anti-Flag and anti-Myc antibodies, respectively. PHR2, photolyase homologous region of CRY2; CCE2, CRY2 C-terminal extension. The cells were treated with blue light (+ Blue; 100 μmol m−2s−1) for 2 h or kept in the dark (-Blue). Arrows show phosphorylated CRY2. The above experiments were repeated three times with similar results. Total ubiquitinated proteins were eluted with 2XSDS sample buffer, denatured at 100 °C for 4 min and subjected to western blot analysis. Anti-ubiquitin antibody (α-Ubq, cat # 14-6078-80, Thermofisher) was used to detect total ubiquitinated proteins, and homemade anti-CRY2 antibody was used to detect CRY2 protein. For FGFP-CRY2 protein purification, the cleared plant lysate were incubated with 50 μl GFP-trap agarose beads (homemade or cat # gta-20, Chromotek) and rotated at 4 °C for 2 h. Beads were pelleted and washed four times with IP buffer (without inhibitors). Proteins were eluted with 2XSDS sample buffer by heating at 100 °C for 4 min and subjected to western blot analysis. Anti-Flag antibody was used to detect FGFP-CRY2 (IP) fusion protein, and anti-ubiquitin antibody was used to detect ubiquitinated CRY2. Statistics and reproducibility For Fig. 1b , n = 16 for WT (dark), n = 15 for WT (red), n = 17 for WT (FR), n = 14 for WT (LD), n = 17 for WT (SD), n = 22 for cry1cry2 (dark), n = 17 for cry1cry2 (red), n = 22 for cry1cry2 (FR), n = 22 for cry1cry2 (LD), n = 22 for cry1cry2 (SD), n = 20 for lrb1lrb2-2lrb3 (dark), n = 25 for lrb1lrb2-2lrb3 (red), n = 25 for lrb1lrb2-2lrb3 (FR), n = 19 for lrb1lrb2-2lrb3 (LD), n = 20 for lrb1lrb2-2lrb3 (SD), n = 18 for cry1cry2lrb1lrb2-2lrb3 (dark), n = 25 for cry1cry2lrb1lrb2-2lrb3 (red), n = 25 for cry1cry2lrb1lrb2-2lrb3 (FR), n = 17 for cry1cry2lrb1lrb2-2lrb3 (LD), n = 18 for cry1cry2lrb1lrb2-2lrb3 (SD). For Fig. 1f , n = 23 for WT (dark), n = 23 for cry1cry2 (dark), n = 20 for lrb1lrb2-2lrb3 (dark), n = 20 for cry1cry2lrb1lrb2-2lrb3 (dark), n = 20 for WT (blue), n = 25 for cry1cry2 (blue), n = 20 for lrb1lrb2-2lrb3 (blue), n = 25 for cry1cry2lrb1lrb2-2lrb3 (blue). For Fig. 1h , n = 21 for WT (dark), n = 24 for lrb1lrb2-2lrb3 (dark), n = 20 for cop1-4 (dark), n = 25 for lrb1lrb2-2lrb3cop1-4 (dark), n = 26 for WT (blue), n = 15 for lrb1lrb2-2lrb3 (blue), n = 23 for cop1-4 (blue), n = 19 for lrb1lrb2-2lrb3cop1-4 (blue). For Fig. 6b , n = 25 for all fluence rates, except n = 21 for WT (30 μmol m −2 s −1 ), n = 24 for cry1cry2 (0 μmol m −2 s −1 ), n = 21 for FGFP-CRY2 (30 μmol m −2 s −1 ). For Supplementary Fig. 1d , e , n = 18 for WT, n = 15 for cry1cry2 , n = 17 for lrb1lrb2-2lrb3 , n = 15 for cry1cry2lrb1lrb2-2lrb3 . For Supplementary Fig. 2b , n = 25 for all, except n = 24 for Myc-LRB2/lrb1lrb2-1lrb3 #61. For Supplementary Fig. 2d , n = 20 for WT (Dark), n = 20 for cry1cry2 (Dark), n = 25 for lrb1lrb2-2lrb3 (Dark), n = 21 for FGFP-LRB2/lrb1lrb2-2lrb3 #5 (Dark), n = 20 for FGFP-LRB2/lrb1lrb2-2lrb3 #8 (Dark), n = 20 for FGFP-LRB2/lrb1lrb2-2lrb3 #17 (Dark), n = 25 for all genotypes in blue. 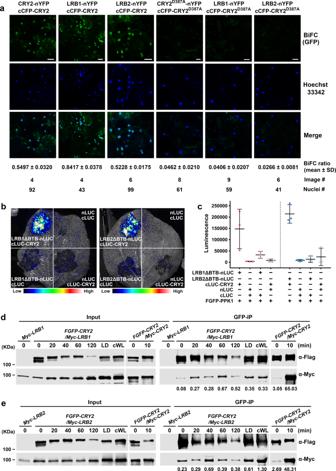Fig. 4: LRBs interact with CRY2 in vivo. aConfocal microscopic images showing BiFC signals of indicated protein pairs transiently expressed inArabidopsisleaves. The Hoechst 33342 (which is used to stain the nuclei) and GFP (BiFC) signals are shown. The relative intensity of CRY2/LRB interaction was presented as BiFC ratio, calculated as BiFC ratio = [GFP intensity]nuclei/ [Hoechst 33342 intensity]nuclei. BiFC ratio (mean ± SD), total number of quantified images and nuclei are shown blow the images. CRY2D387A, photo-insensitive CRY2, is used as the negative control. Scale bars, 10 μm.bSplit-luciferase complementation assays showing the interactions of LRB1 and CRY2 or LRB2 and CRY2 in tobacco. Indicated split-LUC protein pairs were transiently co-expressed inN. benthamianawith FGFP-PPK1. LRB1ΔBTB, LRB1 with deletion of BTB domain (143-212 aa); LRB2ΔBTB, LRB2 with deletion of BTB domain (145-250 aa).cQuantification of split-luciferase complementation assays shown in (b). Data was shown as mean ± SD (n= 3 individual experiments).d–eCo-immunoprecipitation assays showing the interactions of LRB1 and CRY2 (d) or LRB2 and CRY2 (e) inArabidopsis. 7-day-old seedlings expressing Myc-LRB or co-expressing FGFP-CRY2 and Myc-LRB were grown in the dark and then treated with blue light (100 μmol m−2s−1) for the indicated time, or grown in long days (LD, 16 h light/ 8 h dark) and continuous white light (cWL). Plant extracts were immunoprecipitated by GFP-trap beads. The IP and co-IP products were detected with anti-Flag and anti-Myc antibodies, respectively. Co-IP experiments of 7-day-old seedlings co-expressing FGFP-CRY2 and Myc-CRY2 were performed in parallel as positive controls. The relative interaction intensity of CRY2/LRB or CRY2/CRY2 is calculated by [Co-IP intensity] / [IP intensity] and shown blow the immunoblots. The above experiments were repeated twice with similar results. 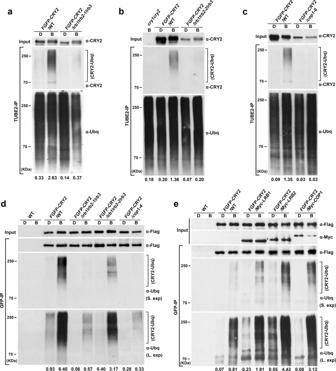Fig. 5: LRBs and COP1 are both required for CRY2 ubiquitination. Immunoblots showing the ubiquitination of FGFP-CRY2 in indicated genotypes. 7-day-old etiolated seedlings constitutively expressing FGFP-CRY2 in indicated genotypes were pretreated with MG132 and kept in the dark or exposed to 30 μmol m−2s−1of blue light for 5, 10, and 15 min. The blue light treated samples (5, 10, and 15 min) were pooled together while performing immunoprecipitation for (a–e).a–cTotal ubiquitinated proteins were purified by TUBE2-conjugated beads. Immunoprecipitated proteins were analyzed by immunoblots probed with anti-ubiquitin antibody (α-Ubq) or anti-CRY2 antibody (α-CRY2). The extent of CRY2 ubiquitination was shown below the immunoblots, calculated as [CRY2-Ubq intensity]IP/[Ubq intensity]IP.d–eFGFP-CRY2 proteins were purified with GFP-trap beads. Immunoprecipitated proteins were analyzed by immunoblots probed with anti-ubiquitin antibody (α-Ubq), anti-Flag antibody (α-Flag) or anti-Myc antibody (α-Myc) for detecting epitope-tagged proteins. The extent of CRY2 ubiquitination is calculated as [CRY2-Ubq intensity]IP/[Flag intensity]IPwith the short exposure immunoblots and shown below the immunoblots. S. exp or L. exp: short or long chemiluminescence exposures of immunoblots. D, dark treatment; B, blue light treatment. The above experiments were repeated at least twice with similar results. 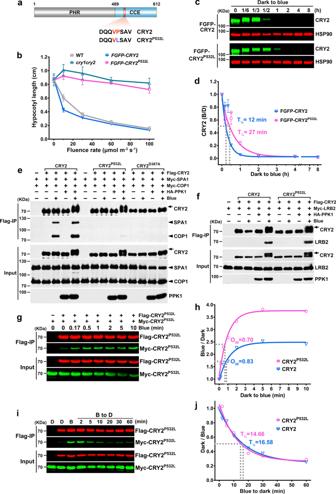Fig. 6: LRBs and COP1 interact with different structural elements of CRY2. aA schematic diagram depicting the CRY2P532Lmutation. PHR, photolyase homologous region; CCE, CRY C-terminal extension; DQQVPSAV, VP motif in CRY2; numbers, amino acid positions.bHypocotyl length of 6-day-old seedlings of indicated genotypes grown under blue light of different light intensities. Data were shown as mean ± SD.cImmunoblots showing degradation of FGFP-CRY2 or FGFP-CRY2P532Lin 7-day-old etiolated seedlings irradiated with blue light (100 μmol m−2s−1) for the indicated time. Immunoblots were probed with anti-CRY2 and anti-HSP90 antibodies.dQuantitative analysis of CRY2 degradation from immunoblots shown in (c),n= 3 individual immunoblots. The best fitted curves with one phase decay of nonlinear regression were shown. CRY2 (B/D) = [CRY2/HSP90]blue/ [CRY2/HSP90]dark. T1/2indicates the time required for 50% degradation.e–fCo-IP assays showing the lack of CRY2P532L/COP1 interaction (e) and the blue light- and phosphorylation-dependent CRY2P532L/LRB2 interaction (f) in HEK293T cells. Transfected cells were either kept in the dark (− Blue) or treated with 100 μmol m−2s−1blue light for 2 h (+ Blue). CRY2D387Ais used as a negative control. Anti-Flag, anti-Myc or anti-HA antibodies were used for detecting indicated tagged proteins. Arrows indicate phosphorylated CRY2.gCo-IP results showing the photooligomerization of CRY2P532Lin HEK293T cells. Transfected cells were irradiated with blue light (30 μmol m−2s−1) for indicated time. CRY2P532Ltagged with Flag or Myc were detected with anti-Flag and anti-Myc antibodies, respectively.hComparison of photooligomerization kinetics of CRY2 and CRY2P532Lin HEK293T cells. Co-IP (α-Myc) signals was normalized to the corresponding IP (α-Flag) signals, and the dark oligomerization level was set as 1. O50indicates the time required to reach 50% saturation of CRY2 photooligomerization. The best fitted curves with one phase association of nonlinear regression were shown.iCo-IP results showing the dark reversion of CRY2P532Lphotooligomers in HEK293T cells. The cells were treated with 30 μmol m−2s−1blue light for 5 min then moved to the darkness for indicated time.jComparison of the dark reversion dynamics of CRY2 and CRY2P532Lphotooligomers in HEK293T cells. Similar analyses were performed as in (h), except that the oligomerization level in blue was set as 1. T1/2indicates the time required to reverse 50% of CRY2 photooligomers into monomers. The best fitted curves analyzed with one phase decay of nonlinear regression were shown. CRY2 photooligomerization and dark reversion data shown in (h) and (j) were extracted from the published paper15with permission. The above experiments were repeated at least twice with similar results. 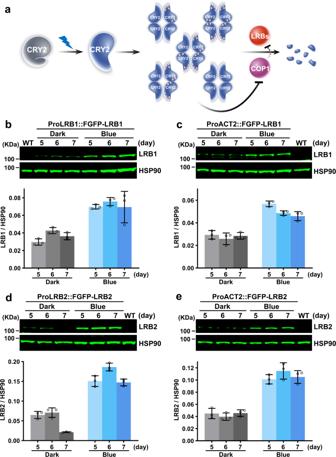Fig. 7: Blue light positively regulates LRBs protein abundance in plants. aA hypothetic model depicting the degradation of CRY2 by LRBs and COP1 E3 ubiquitin ligases. CRY2 exists as inactive monomers in darkness (grey). Upon blue light exposure, CRY2 undergoes photoexcitation, oligomerization, and phosphorylation to become photoactive. Photoactivated CRY2 then were targeted by two distinct E3 ubiquitin ligases, LRBs, and COP1, for degradation. Minus sign in a circle, indicates negative charge; dashed line, indicates a hypothetical mechanism.b–eRepresentative immunoblots (top) and a quantitative analysis (bottom) showing the expression of recombinant LRB proteins in transgenic plants driven by native promoters (b,d) or the ACT2 constitutive promoter (c,e). Seedlings were grown in darkness or continuous blue light (50 μmol m−2s−1) for 5, 6, or 7 days. Proteins were extracted and subjected to western blot analysis. LRBs and HSP90 were detected with anti-Flag and anti-HSP90 antibodies, respectively. HSP90 is used as a loading control. Data were shown as mean ± SD (n= 3 individual immunoblots). The above experiments were repeated at least three times with similar results. Reporting summary Further information on research design is available in the Nature Research Reporting Summary linked to this article.